Nanorings and rods interconnected by self-assembly mimicking an artificial network of neurons Molecular electronics based on structures ordered as neural networks emerges as the next evolutionary milestone in the construction of nanodevices with unprecedented applications. However, the straightforward formation of geometrically defined and interconnected nanostructures is crucial for the production of electronic circuitry nanoequivalents. Here we report on the molecularly fine-tuned self-assembly of tetrakis–Schiff base compounds into nanosized rings interconnected by unusually large nanorods providing a set of connections that mimic a biological network of neurons. The networks are produced through self-assembly resulting from the molecular conformation and noncovalent intermolecular interactions. These features can be easily generated on flat surfaces and in a polymeric matrix by casting from solution under ambient conditions. The structures can be used to guide the position of electron-transporting agents such as carbon nanotubes on a surface or in a polymer matrix to create electrically conducting networks that can find direct use in constructing nanoelectronic circuits. Interconnected molecular systems based on well-defined one-dimensional (1D) and two-dimensional (2D) nanostructures are elusive architectures, which have been proposed as the future basis for nanoelectronic circuits [1] . The latter can act as either logic gates or molecular wires for the transport of individual electrons, photons or magnetic moment in a similar way as observed for natural networks of neurons that serve as the basis for information processing and storage in the brains of living organisms [2] , [3] , [4] , [5] , [6] . However, current approaches for developing molecularly interconnected networks mainly rely on covalent chemistry [7] , [8] . Self-assembly as a tool to form long-range interconnected 1D- or 2D-nanostructures with tuneable optical, electrical and magnetic properties may represent a possible solution towards the mass production of molecular circuits. In such a case, the fabrication of nanostructures would completely rely on spontaneous bottom-up processes depending on different factors: geometry and chemical nature of the building blocks, and their intermolecular forces (that is, Coulombic, van der Waals, dipolar and π–π ) [9] , [10] , [11] , [12] , [13] , [14] , [15] , [16] . The chemical fine tuning of the selected building blocks is an interesting approach, which may give rise to selective formation of interconnected nanoarchitectures after self-assembly. The tailored formation of self-assembled supramolecular nanotubules based on stacked, oligomeric toroids making use of a wedge-like geometry of a polyaromatic molecular synthon aggregated through π -interactions has been reported [17] . Similarly, interconnected pairs of rings (although not in a network fashion) have been constructed using the complementarities of nucleic acid bases in DNA strand-based rotaxanes, taking advantage of the axle rotational flexibility of the chain [18] . In both aforementioned examples, important phenomena that occur in nature are structurally mimicked: the cytoplasmic microtubules [19] and the intracellular hairpin loops [20] from RNA. Such nanostructures may have the potential to be tailored into larger networks with possible applications in the transfer of information (for example, in the form of electricity) and neural network computation [21] , [22] . Structures with analogous architectures have also found wide ranging, emerging applications as components of wave-guiding photonic integrated devices for optical vortex emitters [23] , plasmonic sensing platforms [24] and microtoroid resonators [25] . However, the possibility to translate molecular properties of building blocks capable of self-assembly leading to extended, interconnected networks of rings and rods under ambient conditions has been elusive to date. Such a successful strategy would significantly boost the development of new electronic devices under attractive conditions. Therefore, we designed small molecular building blocks whose self-assembly, electrochemical and magnetic properties may be easily fine-tuned with the ultimate aim to form interconnected networks at the nano/microscale level. To meet this challenging task, we set out to use mono- and bimetallic complexes based on readily available Schiff base ligands, which show structural modularity and thus easy fine tuning of their self-assembly properties [26] , [27] , [28] . In a recent contribution [29] , we reported on the extremely strong self-assembly behaviour of bimetallic bis-Schiff base complexes incorporating aldimine fragments. The self-assembly was mainly mediated by very strong intermolecular Zn–O coordinative patterns, π -interactions and geometric and steric characteristics. However, ketimine-based Schiff base ligands and complexes present more advantages compared with their aldimine counterparts and represent ideal building units from a stability and chemical point of view [30] , [31] . Their chemical structure allows for an easy modulation of their molecular symmetry, shape, flexibility, aromaticity and charge distributions, which, upon combination, have a crucial role in programmable self-assembly and thus configurable 2D and three-dimensional (3D) geometries [32] , [33] , [34] . Additionally, their intermolecular interactions can be also modified by using solvents with different dielectric constants, whereas their electrochemical and magnetic properties can be easily modified by incorporating different metal centres in the Schiff base structures. Here we describe how these Schiff base synthons are effectively used to provide an interesting solution for directed self-assembly leading to unique and defined artificial networks that are interconnected in a neural form; this directed self-assembly is also demonstrated to serve as a template for the collinear alignment and interconnection of carbon nanotubes such that the network’s conductivity is significantly enhanced. Preliminary studies Structural modifications at different positions of the Schiff base scaffold (blue part in molecule 1 Fig. 1 ), in combination with an appropriate selection of the solvent (dichloromethane, DCM; tetrahydrofuran, THF; or toluene) allowed the construction of self-assembled nanostructures with different morphologies ( Fig. 1 and Supplementary Fig. S1 ) from drop-cast solutions. The intermolecular interactions present in this type of Schiff base building block may be the result of various possibilities including intermolecular M–O coordination patterns, van der Waals and/or Coulombic anisotropic interactions with different possible orientations controlled by the dielectric properties of the solvents used [35] . 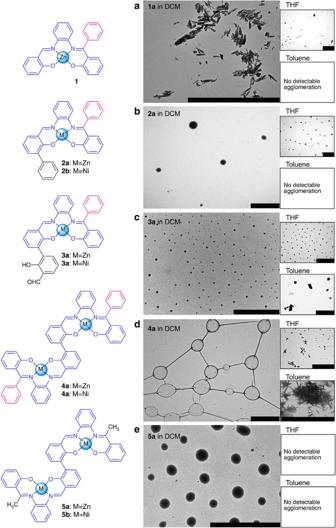Figure 1: Different Schiff base systems studied. Compounds (1–5) are shown at the left and the metal centres used are indicated in each case. In blue, the basic molecular scaffold used as template for the Schiff base complexes; in black and magenta, structural motifs incorporated to fine-tune the self-assembly behaviour of the complexes. The obtained transmission electron microscopy (TEM) images (after solvent evaporation) are shown at the right (panelsa–e) for each compound with the type of the solvent medium indicated. In micrographs, M=Zn; for M=Ni, seeSupplementary Fig. S1. Scale bars for TEM images are 5 μm. Figure 1: Different Schiff base systems studied. Compounds ( 1 – 5 ) are shown at the left and the metal centres used are indicated in each case. In blue, the basic molecular scaffold used as template for the Schiff base complexes; in black and magenta, structural motifs incorporated to fine-tune the self-assembly behaviour of the complexes. The obtained transmission electron microscopy (TEM) images (after solvent evaporation) are shown at the right (panels a – e ) for each compound with the type of the solvent medium indicated. In micrographs, M=Zn; for M=Ni, see Supplementary Fig. S1 . Scale bars for TEM images are 5 μm. Full size image Morphological analysis First, the nanoscopic self-assembly of the (mono) Zn complex 1 was considered by using transmission electron microscopy (TEM). As may be expected for this complex, self-aggregated nanosized flakes were spotted regardless of the solvent used ( Fig. 1 ). These findings are in agreement with the similar complexes previously reported by our group [36] . Next, mononuclear complexes 2a (M=Zn) and 2b (M=Ni) were assessed; these complexes comprise an additional phenyl moiety in an attempt to favour nanoscopic aggregation behaviour through (additional) π -interactions. In the solid state, the compound 2a forms dimeric structures due to the aforementioned intermolecular Zn–O interactions ( Supplementary Fig. S2 ). Homogeneous nanosized quasi-spherical particles were formed from DCM. Surprisingly, compound 2b , which contains a Ni instead of Zn metal centre, also formed well-defined nano- to micro-sized spherical particles ( Supplementary Fig. S1 ). This is an interesting observation, as intermolecular Ni–O interactions in these Schiff base complexes are not very likely as a result of the metal centre being coordinatively saturated. These findings thus suggest that the self-assembly for compounds 2a and 2b is mainly controlled through another mechanism principally based on intermolecular forces other than coordinative M–O bonds. To further investigate the nature of the primary supramolecular interactions involved and gaining more insight how to conceive more complex nanostructures, the presence of polar groups able to mediate intermolecular H-bonding was probed. Compounds 3a and 3b comprising a free phenol and an aldehyde group were subjected to TEM analysis under comparable conditions ( Fig. 1 and Supplementary Fig. S1 ) and evaluated. From their drop-cast solutions analysed by TEM a similar self-assembly into spherical particles was observed, where the size of the aggregates was the only morphological variation compared with those formed with 2a and 2b . On the other hand, if toluene was used as a medium, nanocrystals were observed throughout the sample, which may be the consequence of their reduced solubility in this solvent. Based on the above, it seems that the self-assembly of this family of complexes is driven by van der Waals and π -interactions, and to a much lesser extent by coordinative M–O or H-bonding. Therefore, the incorporation and multiplication of aromatic groups at particular positions in these systems may provide improved molecular self-assembly motifs that can accommodate the formation of two- or three-dimensional nanostructures. Additionally, the control in the possible molecular conformations and their steric requirements should positively contribute to the enhancement of intermolecular self-assembly processes mediated by geometric factors, vectorial short-range interactions and viable combinatorial arrangements [37] . The latter type of self-assembly may be feasible in the case where the individual building units comprise of two bis-Schiff base complexes within the same molecule (for example, Fig. 1 , compounds 4 and 5 ). The use of such building blocks with a rotationally free axle was hence believed to exert a directional effect on the overall association process as a function of the dielectric constant of the solvent used and consequently giving a tool to modulate the resulting nanoarchitectures. To our delight, when tetrakis–Schiff base complexes derived from scaffold 4 were drop-cast from DCM, the formation of interconnected ring-shaped nanoarchitectures was observed with an external diameter interval of 2.105 μm±181 nm and a rim-thickness interval of 138 nm±11 nm (α=0.05, N =42). The rings observed presented long-range interconnections consisting of molecularly highly ordered nanorods (determined by electron diffraction, discussed later) with a thickness of 200 nm±16 nm (α=0.05, N =53) and lengths ranging from hundreds of nanometres up to 15 μm ( Fig. 1 , see Supplementary Figs S3–S5 for full-size images and high-amplification details). Interestingly, the networks could be preserved over large areas (above 300 × 300 μm 2 ). The interconnected structures are reminiscent of networks of neurons occurring in living organisms, where the soma could be represented by the rings and the dendrites and axon by the rods. The formation of this unique interconnected network of nanorings and 1D-nanorods with high length-to-thickness ratios was only possible from DCM. When THF was used, short nanosized strings were observed, wheras nanocrystals were obtained from toluene. In general, the directional vectors of the rods were orthogonal to the rings’ tangent at the ring–rod junction point. The diameter of the ring was also dependent on the hydrophobicity of the supporting surface, with higher hydrophobicity leading to smaller rings. High-angle annular dark field TEM images, confocal laser scanning microscopy and real-time monitoring of the ring formation process at the liquid-solid interface ( Fig. 2 , Supplementary Figs S6 and S7 ) through environmental scanning electron microscopy coupled with energy dispersive X-ray spectroscopy microanalysis demonstrated that after the drop-casting procedure, the complex was only present in the nanostructures; this indicates that also self-assembly processes are occurring in solution. Analogously to the observations for compounds 2 and 3 , the self-assembly mechanism for systems 4 might be related to the molecular shape and to the occurrence of π -interactions possibly modulated by the magenta phenyl group in Fig. 1 , rather than intermolecular forces based on Zn–O or H-bonding interfaces, as both Ni-based 4b and the precursor ligand scaffold ( 4 : no metal) also formed the same structures when drop-cast from DCM ( Supplementary Fig. S1 ). To test this hypothesis, the substitution of the magenta phenyl group in 4 by smaller non-aromatic fragments would have to significantly alter the self-assembly process. Indeed, this was supported when methyl-containing complexes 5a and 5b were used, and no rings or rods could be detected under similar conditions ( Fig. 1 , see also Supplementary Figs S4 and S5 , for full-size and high-amplification TEM comparison between selected compounds 4a and 5a ). 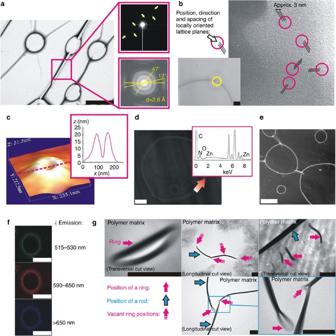Figure 2: Characterization of the structures on surfaces and in a polymer matrix. (a) TEM micrograph obtained from DCM showing a network structure (insets show electron diffraction and fast Fourier transform–FFT–patterns from a typical rod as the one shown in the figure, arrows indicate diffraction spots); scale bar is 5 μm. (b) High-resolution TEM (HR-TEM) of a ring section; left/right=low/high magnification of the zone indicated; right, parallel black lines indicate the position, direction and spacing of locally oriented lattice planes enclosed by the magenta circles; scale bar of inset at left is 400 nm. (c) Atomic force microscopy (AFM) 3D surface profile image of one of the ring structures, the height of rods is apparently smaller than the sensibility of the device. The inset shows the height measured as a function of thexcoordinate along the dashed magenta line. (d) Environmental scanning electron microscopy (ESEM) image of a ring after real-time formation follow-up (scale bar is 1 μm) and energy dispersive X-ray spectroscopy (EDX) microanalysis carried out during the ESEM monitoring. (e) High-angle annular dark field TEM (HAADF-TEM) image of the structures, bright regions are the complex; scale bar is 2 μm. (f) Confocal laser scanning microscopy (CLSM) image of a ring excited at 488 nm, and emitting at three different wavelength intervals (top=515–530 nm, centre=590–650 nm and bottom>650 nm); scale bars, 5 μm. (g) Nanorings interconnected by rods from4aembedded in a polycarbonate matrix (longitudinal and transversal cut views) observed by TEM; scale bars, 1 μm; regions containing rings, rods or vacant ring positions are indicated by the respective arrows. Figure 2: Characterization of the structures on surfaces and in a polymer matrix. ( a ) TEM micrograph obtained from DCM showing a network structure (insets show electron diffraction and fast Fourier transform–FFT–patterns from a typical rod as the one shown in the figure, arrows indicate diffraction spots); scale bar is 5 μm. ( b ) High-resolution TEM (HR-TEM) of a ring section; left/right=low/high magnification of the zone indicated; right, parallel black lines indicate the position, direction and spacing of locally oriented lattice planes enclosed by the magenta circles; scale bar of inset at left is 400 nm. ( c ) Atomic force microscopy (AFM) 3D surface profile image of one of the ring structures, the height of rods is apparently smaller than the sensibility of the device. The inset shows the height measured as a function of the x coordinate along the dashed magenta line. ( d ) Environmental scanning electron microscopy (ESEM) image of a ring after real-time formation follow-up (scale bar is 1 μm) and energy dispersive X-ray spectroscopy (EDX) microanalysis carried out during the ESEM monitoring. ( e ) High-angle annular dark field TEM (HAADF-TEM) image of the structures, bright regions are the complex; scale bar is 2 μm. ( f ) Confocal laser scanning microscopy (CLSM) image of a ring excited at 488 nm, and emitting at three different wavelength intervals (top=515–530 nm, centre=590–650 nm and bottom>650 nm); scale bars, 5 μm. ( g ) Nanorings interconnected by rods from 4a embedded in a polycarbonate matrix (longitudinal and transversal cut views) observed by TEM; scale bars, 1 μm; regions containing rings, rods or vacant ring positions are indicated by the respective arrows. Full size image Self-assembly in a polymer matrix The self-assembled structures formed by 4a from DCM were also formed inside 50 μm thickness polymeric films prepared by casting solutions of both 4a and a bis-phenol-A based polycarbonate from DCM. Transversal and longitudinal cuts of the films containing the complex 4a were analysed through TEM and confirmed that the interconnected structures could be retained as 3D arrangements inside solid matrices ( Fig. 2g ). Compared with their counterparts formed on a flat surface, the ring diameter in the polymer films varied from a hundred nanometres to a couple of micrometres, whereas the rods appeared thicker. Importantly, the interconnectivity remained basically intact, showing this self-assembly process having potential for applications in material science and polymer based nanoelectronics. In silico study It is important to mention here that the spontaneous formation of rings by self-assembly has been scarcely reported. Most of the reported structures follow formation mechanisms derived from de-wetting processes in which either the spontaneous formation of pinholes, 2D bubbles, the concentric accumulation of material mediated by local capillarity (coffee-stain effect) or Marangoni-flow engineering produce rings on flat surfaces [38] , [39] , [40] , [41] , [42] , [43] , [44] . However, none of the latter mechanisms can explain the formation of the rings for derivatives 4 that are interconnected in a neural network fashion both on flat surfaces and inside a polymeric matrix. Therefore, a two-level in silico study was carried out in order to determine the kinetic and thermodynamic feasibility for this generation of molecules to form highly ordered and extended structures. Density functional theory (DFT) calculations have been performed with complex 4a to evaluate the lowest energy and most favourable molecular geometry of the building unit ( Supplementary Fig. S8 ) and the charge distribution ( Supplementary Fig. S9 and Supplementary Table S1 ). In this manner, it could be possible to estimate intermolecular binding energies and thus, the most stable mutual molecular orientations upon self-assembly ( Supplementary Note 1 ). However, such electronic level calculation is a very computationally intensive task, limited to systems containing (depending on system complexity) up to several hundreds of atoms. Therefore in a second phase, the evolution of assembled systems containing up to 450 molecules of 4a were studied with molecular dynamics (MD) simulations using previously optimized geometry and electrostatic atomic charges derived from DFT calculations. Compound 4a may be represented by a ‘wedge’ that is spatially defined by the angle (102° in equilibrium) between both pairs of Schiff base units (for example, biphenyl spacer) with the ends of the wedge pointing to the metallic centres in 4a ( Fig. 3a ) and the centre of the wedge designated as ‘tip’. The side to which the tip points is defined as ‘face’ and the opposite side as ‘back’. 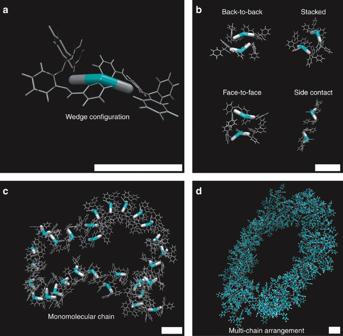Figure 3:In silicostudy of4ain multimolecular systems. (a) Wedge designation for4a. (b) Most favourable bimolecular configurations. (c) Formation of a circular structure from a mononuclear string. (d) Full ring structure from a multimolecular thick chain. Scale bars, 10 Å. Figure 3: In silico study of 4a in multimolecular systems. ( a ) Wedge designation for 4a . ( b ) Most favourable bimolecular configurations. ( c ) Formation of a circular structure from a mononuclear string. ( d ) Full ring structure from a multimolecular thick chain. Scale bars, 10 Å. Full size image Due to this geometry, molecules of 4a have anisotropic binding ability. The most stable intermolecular orientations were found to be (from stronger to weaker) ‘back-to-back’, ‘stacked’, ‘face-to-face’ and those referring to a ‘side contact’ (see Fig. 3b , Supplementary Note 2 and Supplementary Figs S10–S12 ). A synergistic contribution of all these possible orientations might occur during the formation of the self-assembled nanostructures in solution and solid phase. However, the computational data have shown that electrostatic interactions have an important role in the last three configurations ( Supplementary Table S2 ), thus making it possible to control the structure of multimolecular systems in solution by changing the dielectric properties of the solvent. As a result of the mutual orientation of the molecules and their binding energy anisotropy, it is kinetically favourable for 4a to form chain-like structures with significant flexibility ( Supplementary Fig. S13 ). These molecular chains can easily relax the conformational stress by local flipping of the orientation and therefore develop non-uniform structures. Curiously, these aggregated systems have the tendency to form maximally closed configurations, especially at the open ends of the chain and in surface layers. In combination with the anisotropic binding energy profile of 4a , spontaneous fluctuations of molecular orientation cause local ordering leading to bending of entire sections to one side thus forming ring-like structures either as single monomolecular chains ( Fig. 3c ) or multichain arrangements ( Fig. 3d ). The overall arrangement of these assembled structures and the high amount of surface molecules with their ‘tip’ oriented outside the multichain arrangement ( Supplementary Fig. S14 ) improves the bending capability and helps to stabilize arc-like structures ( Supplementary Fig. S15 ) without having these collapsing into a droplet ( Supplementary Note 3 ). This type of geometric arrangement in similar wedge-like aromatic subunits has previously demonstrated to have high effectiveness in stabilizing toroidal and nanotubular assemblies. [17] Interestingly, full rings simulated from bent multichain assemblies (rim thickness of several layers of molecules) did not change their arrangement once the ring structure was formed because their total kinetic and potential energies already fluctuated around equilibrium values ( Supplementary Fig. S16 ). In situ studies In addition, an extensive in situ study was carried out to elucidate a probable formation mechanism of these interconnected ring-shaped assemblies. Considering different geometric parameters such as statistical dimensions from TEM ( Supplementary Fig. S3 ), intermolecular distances from scanning transmission electron microscopy (STEM) electron diffraction at the rods (2.6 nm, from Fig. 2a ) and from high-resolution TEM (HR-TEM) at the rings (3 nm, from Fig. 2b and Supplementary Fig. S17 ) and the hydrodynamic diameter of 4a in CD 2 Cl 2 (19.68 Å) calculated from DOSY ( Supplementary Fig. S18 ), it can be assumed that the intermolecular distance remains approximately the same in the rings as in the rods. With this information, the width of the rods ( W ), the rims transversal diameter/circumference/area ( D TR / C TR / A TR ) and the rings external/internal circumference ( C RE / C RI ) in terms of number of molecules consecutively aligned along the measured parameter ( Fig. 4 ) using a toroidal approximation for the shape of the ring may also be derived. Following that basic approximation, we estimated that an average ring should contain about 1.2 × 10 7 –2.0 × 10 7 molecules in a densely packed model. Dynamic light scattering (DLS) measurements of 4a in DCM clearly showed the presence of three differently sized species, with radii intervals of 10–40 Å, 80–400 nm and 4.2–5.6 μm, respectively. These species can be attributed to free molecules and differently sized assemblies. If the largest agglomeration is approximated to a hollow unilamellar vesicle model, it is possible to estimate a size corresponding to 5.5 × 10 7 –1.3 × 10 8 molecules. This suggests that in solution also assemblies with similar dimensions can be present as observed on flat surfaces. The tendency of 4a towards self-assembly was observed regardless of the concentration of the DLS sample in the interval of 1 × 10 −6 M to 1 × 10 −4 M. This was also confirmed by TEM, when drop-cast solutions prepared in the latter concentration interval provided, in basic terms, similar structures. On the contrary, more diluted solutions afforded no observable assemblies and higher concentrations derived into dense aggregates ( Supplementary Fig. S19 ). The filtration of samples through filters with a pore diameter of 50 nm did not affect the size and population densities of the signals observed in DLS. Therefore, the formation of the aggregates in DCM should follow a dynamic and reversible self-assembly process derived from the wedge-like molecular conformation and predominantly be based on van der Waals, Coulombic and aromatic intermolecular interactions [45] , [46] . 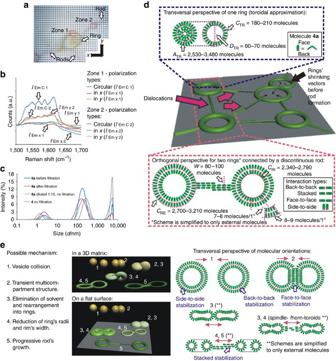Figure 4: Studies for the determination of the possible formation mechanism. (a) Nanostructures analysed by surface-enhanced Raman scattering (SERS) microscopy; scale bars forxandyare 10 μm. (b) SERS emission spectra from the different zones and at three different exciting light polarization conditions: circular, normal (x) and orthogonal (y) polarization. Zone 1, spectra obtained when the laser spot was addressed towards the rim of a ring; zone 2, spectra when the laser was exciting a region with a rod. (c) Dynamic light scattering (DLS) size distribution by intensity in DCM of a4anon-filtered solution (0.35 mM),4aafter filtration of the solution,4anon-filtered and diluted 1:10 (0.035 mM) and a control experiment with ligand4(0.35 mM). (d) Possible molecular orientation vectors in the different structures and estimation of the average number of molecules involved therein, using a toroidal approximation mathematic model. (e) Proposed mechanism of formation for the interconnected rings in both, flat surfaces and 3D polymeric matrices indicating the possible molecular orientation vectors during the process. Figure 4: Studies for the determination of the possible formation mechanism. ( a ) Nanostructures analysed by surface-enhanced Raman scattering (SERS) microscopy; scale bars for x and y are 10 μm. ( b ) SERS emission spectra from the different zones and at three different exciting light polarization conditions: circular, normal ( x ) and orthogonal ( y ) polarization. Zone 1, spectra obtained when the laser spot was addressed towards the rim of a ring; zone 2, spectra when the laser was exciting a region with a rod. ( c ) Dynamic light scattering (DLS) size distribution by intensity in DCM of a 4a non-filtered solution (0.35 mM), 4a after filtration of the solution, 4a non-filtered and diluted 1:10 (0.035 mM) and a control experiment with ligand 4 (0.35 mM). ( d ) Possible molecular orientation vectors in the different structures and estimation of the average number of molecules involved therein, using a toroidal approximation mathematic model. ( e ) Proposed mechanism of formation for the interconnected rings in both, flat surfaces and 3D polymeric matrices indicating the possible molecular orientation vectors during the process. Full size image From surface-enhanced Raman scattering (SERS) microscopy using circularly, normally ( x ) and orthogonally ( y ) polarized excitation, it was observed that the emission spectra at the rings and rods strongly depended on the polarization angle in the light of the laser applied. This indicates that the molecules present in both types of structures should be preferentially oriented in certain directions. In Fig. 4a,b , the decrease in the emission spectra peak size is the evidence of a reduced fraction of molecules that are coherent with the angle of polarization, whereas a relative increase in the signal would indicate a higher density of molecules with collinear orientation vectors. From the latter results and based on the previously described in silico studies, we propose that the ‘back’ of the molecules at the rim of the rings are radially oriented towards the centre of the rim whereas the inner layers of molecules should be present in different combinations of concentrically arranged intermolecular configurations. This combined configuration may in turn provide overall stabilization to the circular structures. Simultaneously, the rods should mainly contain molecules with the same orientation vector dominant at the connection point between the ring and the rod (producing electron diffraction spots as in Fig. 2a ). The HR-TEM micrograph in Fig. 2b taken from a discontinuous section in a ring segment shows that having multiple orientations of arranged layers within the ring body is most likely (see examples of locally oriented lattice planes indicated in the figure). From this viewpoint, and comparing with the DLS results we believe that a possible formation mechanism starts with the solvent (DCM) stabilizing the formation of spherical hollow vesicles. During the elimination of DCM from the system, the vesicles collision probability is increased, which results into a higher degree of vesicle inter-adherence and creation of transient structures morphologically similar to multi-compartment micelles [47] , ( Supplementary Fig. S6 ), which might be stabilized by face-to-face interactions. Subsequently, progressive elimination of the solvent simultaneously promotes a reduction in the vesicles radii and a flattening process of the vesicles shapes due to molecular migration from the center of the vesicles towards the edges through spindle-like and horn-like toroid intermediates thus generating rings at the end of the process ( Fig. 4e ). During the ring formation and size reduction process, the oppositely oriented molecules present at a multi-vesicular contact point self-organize following the same molecular orientation vectors as present at the tangential point of the local curvature. In this way, rod growth takes place from available material present at the external edge of the rings, and eventually this provides an equilibrium between ring size and rod length, yielding rods with stacked molecules in segments of opposite orientation. This would explain the presence of rods with an epitaxial-like structure intermittently disrupted by ‘dislocations’ ( Fig. 2a and Supplementary Fig. S4 ). The shear stress forces exerted from the nanorings during their formation on flat surfaces may also contribute to these irregularities, thus resulting in either ladder-like rods or structures with disrupted continuity. In addition, the stability of the rods with such irregularities could be the result from side-to-side intermolecular interactions and from the flexibility imposed by the molecular axle represented by the biphenyl fragments in the tetrakis–Schiff base systems. Real-time formation of the rings followed in video mode by controlled solvent evaporation through cryo-environmental scanning electron microscopy also supported this formation mechanism ( Supplementary Fig. S7 ). Application of the concept Finally, the possibility for the network to serve as an effective structure for transmitting electrical information over longer distances was explored. The structures themselves, neither on a surface nor embedded in a solid polycarbonate matrix, demonstrated to be electrically conductive. Therefore, the network was used as a positional template for a compatible electron-transporting agent such as multiwalled carbon nanotubes (MWCNT) both on a surface as well as in a solid polycarbonate matrix. A drop-cast solution of 4a containing MWCNTs (mean length 1.04 μm, outer diameter 13–16 nm) in DCM analysed by TEM showed a long-range (above 300 × 300 μm 2 ) collinear self-assembly of the nanotubes onto the rods and rings in the network ( Fig. 5b ). Moreover, by using shorter nanotubes (length=100–700 nm, outer diameter=15–42 nm), it was possible to form individual rings made of nanotubes ( Fig. 5c ). Such ordering effect was not observed from drop-cast DCM solutions containing only MWCNTs, where (expected) random arrangements where obtained ( Fig. 5f ). Subsequently, bis-phenol-A polycarbonate films of 50 μm thickness containing MWCNTs and complex 4a were prepared in the same way as described earlier and further compared with their counterparts prepared only from MWCNT. A comparative TEM analysis of transversal cuts from the latter films confirmed that the strong tendency of the nanotubes to remain distributed in a random fashion in a solid polymer matrix–containing only MWCNT–( Fig. 5d ) was efficiently prevented when the films also contained self-assembled complex 4a . Transversal cuts from films containing both MWCNTs and 4a showed the presence of rod structures from the complex and carbon nanotubes, which were consecutively aligned and collinear to the assemblies formed by 4a . In this sense, the strong self-assembly tendency of 4a to form interconnected networks from cast solutions has mediated the system to the entropically favoured formation of extended collinear networks of interconnected carbon nanotubes over larger areas and volumes. This spatially aligned higher-level superstructure is facilitated by the considerable shape anisotropy of the nanotubes and the rods/rings in the molecular network, thus resulting in entropy-driven directional ordering [43] , [48] . Although this is not the first case of circularly arranged nanostructures (for example, nanoparticles [41] , [49] , [50] , [51] , nanorods, [52] , nanowires [53] , carbon nanotubes [54] , [55] ), it represents to our knowledge the first example where self-assembled structures can efficiently address the orientation and interconnection of carbon nanotubes, both in circular structures and in long-range networks, and in a solid polymer matrix. Films containing compound 4a and carbon nanotubes afforded significantly higher electrical conductivities ( σ ) at equivalent loads of MWCNTs when compared with films prepared only from the polymer and nanotubes ( Fig. 5h,i ). It is important to mention that the incorporation of 4a into the polycarbonate matrix did not affect the electrical behaviour of the pure material: sheet–surface conductivity ( σ s ) was preserved in the range of 10 −17 –10 −16 S sq., volumetric conductivity ( σ v ) was kept below 10 −18 S m −1 . However, the incorporation of MWCNT (2–3% vol.) into the pure polycarbonate matrix increased both the sheet and volumetric conductivities to 2.5 × 10 −13 S sq. and 4.7 × 10 −5 S m −1 , respectively. Interestingly, when 4a was also incorporated into the film version containing MWCNTs, σ s increased in seven orders of magnitude (2.6 × 10 −6 S sq., s.d.=2.3 × 10 −7 S sq., N =3), and σ v followed the same tendency in two orders of magnitude (3.1 × 10 −3 S m −1 , s.d.=3.9 × 10 −3 S m −1 , N =3), in comparison with the films prepared only from MWCNTs. The latter observation agrees with the model of self-assembled 3D networks of interconnected carbon nanotubes. 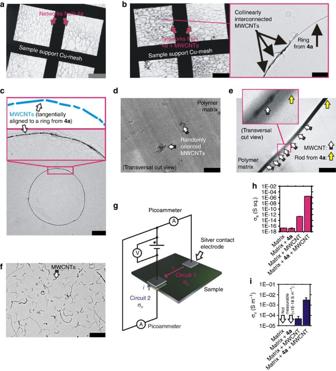Figure 5: Applications of the self-assembled network based on4a. (a) TEM image of a Cu-grid after drop-casting a DCM solution of4a(7 × 10−5M); scale bar, 50 μm. (b) TEM analysis of4a(7 × 10−5M) containing multiwalled carbon nanotubes (MWCNT) at 0.02 mg ml−1after drop-casting from DCM; MWCNT mean length=1.04 μm, diameter=13–16 nm; scale bars, (left to right) 50 μm and 500 nm. (c) Drop-cast DCM solution of4a(1 × 10−5M) and shorter MWCNTs (0.02 mg ml−1); MWCNTs in magnification are green lines; MWCNT length=100–700 nm, diameter=15–42 nm; scale bar, 1 μm. (d) TEM image from transversal cut of a film composed by polycarbonate and MWCNTs (1.52 × 10−2% vol.); scale bar, 500 nm. (e). TEM micrograph from a transversal cut of a polycarbonate film containing4a(0.07% wt.) and MWCNTs (1.52 × 10−2% vol); scale bar, 500 nm. (f). TEM image of MWCNTs, when drop-cast from DCM (0.02 mg ml−1); scale bar, 500 nm. (g) Examples for the circuits used to test the films; circuit 1=measurement of sheet conductivity (σs), circuit 2=measurement of volumetric conductivity (σv). (h) Sheet conductivities for films; error bars are 1 s.d. forN=3; in some cases, error bars are smaller than the width of the bar frame lines. (i) Volumetric conductivities for films; error bars are 1 s.d. forN=3. Forhandi, the four film compositions tested are, from left to right: polycarbonate matrix; polycarbonate+complex4a(0.07% wt); polycarbonate+MWCNT (2% vol. forh, 3% vol. fori); polycarbonate+4a(0.07% wt.)+MWCNT (2% vol. forh, 3% vol. fori). Figure 5: Applications of the self-assembled network based on 4a . ( a ) TEM image of a Cu-grid after drop-casting a DCM solution of 4a (7 × 10 −5 M); scale bar, 50 μm. ( b ) TEM analysis of 4a (7 × 10 −5 M) containing multiwalled carbon nanotubes (MWCNT) at 0.02 mg ml −1 after drop-casting from DCM; MWCNT mean length=1.04 μm, diameter=13–16 nm; scale bars, (left to right) 50 μm and 500 nm. ( c ) Drop-cast DCM solution of 4a (1 × 10 −5 M) and shorter MWCNTs (0.02 mg ml −1 ); MWCNTs in magnification are green lines; MWCNT length=100–700 nm, diameter=15–42 nm; scale bar, 1 μm. ( d ) TEM image from transversal cut of a film composed by polycarbonate and MWCNTs (1.52 × 10 −2 % vol. ); scale bar, 500 nm. ( e ). TEM micrograph from a transversal cut of a polycarbonate film containing 4a (0.07% wt.) and MWCNTs (1.52 × 10 −2 % vol); scale bar, 500 nm. ( f ). TEM image of MWCNTs, when drop-cast from DCM (0.02 mg ml −1 ); scale bar, 500 nm. ( g ) Examples for the circuits used to test the films; circuit 1=measurement of sheet conductivity ( σ s ), circuit 2=measurement of volumetric conductivity ( σ v ). ( h ) Sheet conductivities for films; error bars are 1 s.d. for N =3; in some cases, error bars are smaller than the width of the bar frame lines. ( i ) Volumetric conductivities for films; error bars are 1 s.d. for N =3. For h and i , the four film compositions tested are, from left to right: polycarbonate matrix; polycarbonate+complex 4a (0.07% wt); polycarbonate+MWCNT (2% vol. for h , 3% vol. for i ); polycarbonate+ 4a (0.07% wt. )+MWCNT (2% vol. for h , 3% vol. for i ). Full size image This study shows that it is possible to modulate molecular self-assembly properties of Schiff base scaffolds towards more complex, controlled nanoarchitectures. The unique interconnected, neural-like networks based on 4 generated either on flat surfaces or in solid polymeric matrices can be exploited for example, as a template for positioning a compatible electron-transporting agent such as carbon nanotubes to generate electrically conducting materials with potential direct uses in molecular circuits or nanoelectronic materials. Finally, the possibility to have self-assembled networks consisting of tetrakis–Schiff base complexes incorporating different metals such that their electrochemical, magnetic or optoelectronic characteristics may be tailored without affecting the overall features of the assembled architectures also offers an interesting opportunity in different fields, such as sensoring platforms, integrated circuits and composite materials. Transmission electron microscopy TEM analysis was performed on a JEOL model JEM-1011 electron microscope with an acceleration voltage of 100 keV, 50 micrometre C2 aperture, spot size 3 and variable dose rate. Liquid samples were prepared by drop-casting 0.35 mM solutions (concentration deviations are mentioned in the text) of the corresponding compound (previously dissolved in the selected solvent) on formvar carbon film-covered square mesh copper grids and dried completely for 4 h. Alternatively, samples containing MWCNTs (Nanocyl SA, Sambreville, Belgium and HeJi, Shenzhen, China) were drop-cast following the same procedure. Such samples were prepared by mixing appropriate aliquots from a master batch dispersion of the nanotubes in DCM (previously sonicated for 15 min) with a solution containing 4a in DCM at the concentration tested. Solid samples were embedded in an epoxy-based resin, cured for 72 h at 80 °C, cut with a microtome and fixed on a double copper grid fixation system for analysis. HR-TEM and electron diffraction analysis HR-TEM analysis was performed on a Philips CM200 electron microscope with an acceleration voltage of 200 keV, 50/100 micrometre C2/C3 apertures, spot size 2 and dose rate 30 A cm −2 . HR-TEM electron diffraction was obtained through selected area mode diffraction in a camera length of 700 mm. Electron diffraction analysis by STEM STEM electron diffraction was performed on a Tecnai F30 microscope. The data were obtained with a nanobeam, created by having a defocused STEM probe, with an accelerating voltage of 300 keV, dose rate 1–5 e Å −2 , 10 μm C2 aperture, and the microscope in microdiffraction mode, gun lens 8 spot size 8 for a 50 nm probe on the sample with a quasi-parallel illumination, convergence of 0.2 milliradians. The data were recorded on a CCD camera Gatan 694 MSC 1,024 × 1,024. Sample analysed by STEM electron diffraction were prepared by drop-casting 0.35 mM in DCM solutions of the corresponding compound on formvar carbon film-covered square mesh copper grids and dried completely for 4 h. Environmental scanning electron microscopy Microscopic analysis was carried out at 4 Torr, 10 °C and 30 kV using a FEI Quanta microscope with ETD, model 600 coupled to an X-ray microanalyser. Liquid samples were prepared by drop-casting required solutions (0.35 mM in DCM) on a metal slide for wet sampling and completely evaporated prior to analysis. Solid samples were fixed on sample holders without any previous treatment and directly analysed at the microscope. Real-time formation of the rings was followed in video mode from a drop-cast solution of the compound progressively dried by increasing the temperature of the sample from 253.45 K to 283.15 K at 7.9 × 10 −3 to 5.3 × 10 −3 atm. Atomic force microscopy AFM analysis was performed at tapping mode on a molecular imaging model Pico SPM II (Pico+) microscope and processed with WSxM [56] package. Samples were prepared by drop-casting solutions (0.35 mM in DCM) on a planar mica sheet. Confocal laser scanning microscopy Confocal laser scanning microscopy analysis was carried out with a Nikon TE2000-E inverted microscope and an excitation Ar laser beam source of 488 nm. Samples were prepared by drop-casting solutions (0.35 mM in DCM) on a glass slide. SERS microscopic analysis Data were recorded with a Renishaw FT-IR-Raman spectrometer coupled with a confocal microscope (Leica DM 2500) at an excitation wavelength of 633 nm, a laser spot size of 5 μm and 10-s acquisition time. Samples were prepared by drop-casting solutions (0.35 mM in DCM) on 4 mm × 4 mm Klarite (R) SERS gold surface slides. Dynamic light scattering DLS analysis was carried out on a Zetasizer Nano Zs (Malvern Instruments Ltd.) with 532 nm laser radiation source. 1 ml of the corresponding solution (0.35 mM in DCM) was analysed on a standard fluorescence glass cuvette with an optical path length of 1 cm. In silico studies DFT calculations were carried out using SIESTA [57] and ONETEP [58] packages for an efficient minimization of the electronic energy functional. OPUIM package was used to generate pseudopotentials to replace core electrons. Single point k-space sampling and local density approximation in Perdew & Zanger parameterization were used for electron exchange and correlation functional for both packages. GTO6-31 basis in NWCHEM [59] package was used to fit atomic charges to electrostatic potential from all-electronic calculations. MD simulations were performed using LAMMPS [60] package. DREIDING force field was used to describe bonds and van der Waals interactions. DFT 61,62 calculations were carried out using SIESTA and ONETEP packages in a two-step optimization procedure. Both packages efficiently minimize electronic energy functions by expanding the eigenfunctions (corresponding to electronic orbital wave functions) in predefined basis and variation of expansion coefficients. Within SIESTA method valence electrons were expanded in double zeta plus polarization basis set of numerical atomic orbitals. 63 Basis was generated using split-valence method, energy shift was set to 50 meV. Popular for its efficiency and sufficient accuracy in most cases, it allows quite robust geometry optimization. Basis set superposition error arising from relatively small number of basis functions was corrected using counterpoise method. 64 Core electrons were replaced by Troullier–Martins pseudopotentials 65 for faster computation. A cut-off of 300 Ry was used for grid integration. ONETEP package represents electronic orbitals using nonortogonal generalized Wannier functions that are in turn expanded in periodic sinc functions. [58] Due to such choice of basic functions, no basis set superposition error correction is needed and very accurate atomic forces and geometry optimization can be achieved, 66 however much more intensive computation is required than in SIESTA case. Non-orthogonal generalized Wannier function’ radii were set to 8 bohr. Pseudopotentials generated by OPUIM package 67 were used to replace core electrons. For fully converged energies, plain wave cut-off was set to 1,000 eV. Single point k-space sampling and local density approximation in Perdew & Zanger parameterization 68 were used for electron exchange and correlation functional for both packages. Iterative self-consistent calculations were conducted until energy convergence below 50 meV and maximum forces below 50 meV/atom for single molecule and 100 meV/atom for bimolecular complex were achieved. Atomic charges were calculated using Mulliken population 69 and natural bond orbital analysis 70 in ONETEP and by fitting to electrostatic potential from all-electronic calculation using GTO6-31 basis in NWCHEM package for comparison. MD simulations were performed using LAMMPS package. Bonded and van der Waals interactions’ parameters were assigned according to DREIDING force field. 71 To simplify, computation molecule was divided to four connected parts treated as rigid bodies ( Supplementary Fig. S8 ). To eliminate possible atomic overlap due to poor choice of initial positions in the beginning of each simulation, soft interatomic potentials were used for 1,000 steps to displace molecules to safe initial positions. After that NVT ensemble calculations were performed at 300 K during up to 10 7 steps (equivalent to 10 ns). First, single 4a and double molecular complex were placed in a 50 × 50 × 50 Å simulation box and their geometries were optimized first using more robust SIESTA code ( Supplementary Fig. S9 ), than using more precise ONETEP. On the second stage, series of MD simulations of bimolecular complex were performed with one molecule fixed in the middle of the periodic box and initial position and orientation of the other were chosen randomly. Molecular system evolution was simulated during 10 5 time steps (~100 ps). From the final bimolecular structures those where stabilized bimolecular complexes had formed were selected and analysed. Several periodic structures were taken as the starting point for further simulation. In each simulation, molecular system was initiated as a string with free ends 9–64 molecules long, 1 to 9 molecules in cross-section and left at constant volume box under the temperature of 300 K. The segment shown on Supplementary Fig. S15 was mirrored to form a full ring, which was further simulated as a single object ( Fig. 3d ) during additional 10 7 time steps (~10 ns). No structural changes were observed with system’s kinetic and potential energies fluctuating around equilibrium ( Supplementary Fig. S16 ). Preparation of polymer films Polymer films were prepared by casting solutions containing 10% m/v high-purity optical storage media grade Bis-phenol-A polycarbonate (Bayer) and different concentrations of the required molecule (0.01–0.35 mM). The solutions were prepared by dissolving the compounds in anhydrous dichloromethane (purity 99.8%) purified, filtered and dried through a high-throughput solvent purification system. The films were prepared under high-efficiency particulate air-filtered laminar flow conditions. Remaining solvent in the films was eliminated under vacuum and heat (10 mBar, 80 °C). The thickness of the film was controlled to a final value of 50 μm in the solid state. The same protocol was followed for preparing the samples containing multiwalled carbon nanotubes, by also incorporating the desired amount of nanotubes (1.52 × 10 −2 –3% vol.) into the liquid matrix before casting. Electrical characterization of materials Surface and volumetric electrical conductivity of solid films at conductivity values above 10 −6 S (net readout) were determined following the two-point testing method using a Keithley High Performance Digital Multimeter 2000 under automatic voltage sweep mode. Samples with the dimension 6 cm × 6 cm were pre-treated at the measuring contact points with 4 mm width/15 mm spacing thin layer strips of silver ink (Electrodag 1415, Agar Scientific). Surface conductivity of solid films at conductivity values below 10 −6 S (net readout) was determined with a Keithley Model 8009 high resistivity test fixture with integrated Faraday box electrostatic shielding system coupled to a Keithley 6487 Picoammeter/Voltage Source. Film samples with the same abovementioned dimensions were directly analysed within the fixture without any previous treatment at applied voltage of 500 V. Volumetric conductivity measurements were carried out under the same latter conditions. General synthesis and characterization All starting materials were purchased from commercial sources and used without further purification. Elemental analyses were performed at the Unidad de Análisis Elemental of the University of Santiago de Compostela (Spain). All NMR measurements were carried out on a Bruker-400 MHz spectrometer at ambient temperature unless stated otherwise, and chemical shifts are given in parts per million versus TMS. Mass spectrometric and X-ray diffraction data were obtained from the Research Support Unit of the ICIQ and MALDI-TOF mass spectrometric experiments were carried out using pyrene as matrix. Compounds (E)-2-(((2-aminophenyl)imino) (phenyl)methyl) phenol, 72 3,3′-diformyl-2,2′-dihydroxy-1,1′-biphenyl, 73 2-hydroxy-[1,1′-biphenyl]-3-carbaldehyde, 74 2-((E)-((2-((E)-(2-hydroxo-benzylidene)amino) phenyl)imino)(phenyl)methyl)phenoxo Zn complex 1 , 75 3-((E)-((2-((E)-((2-hydroxyphenyl)(phenyl) methylene)amino)phenyl)imino)methyl)-[1,1′-biphenyl]-2-ol (Bis-Schiff base ligand 2 ), complex 2a , 3,3′-bis((E)-((2-((E)-((2-hydroxyphenyl)(phenyl)methylene)amino)phenyl)imino)methyl)-[1,1′-biphenyl]-2,2′-diol (tetrakis–Schiff base ligand 4 ), complex 4a [30] and complex 4b 75 were synthesized using reported methodologies. For X-ray crystallographic structure from 4 see Supplementary Fig. S20 . Synthesis of Bis-Schiff base Ni complex 2b A solution of 2 (100 mg, 0.21 mmol) in 5 ml of CHCl 3 and Ni(AcO) 2 ·4H 2 O in 5 ml of MeOH was stirred for 18 h. A brownish suspension was formed, the solid was filtered and washed with MeOH. Brownish solid, 101 mg, 92%. 1 H NMR (400 MHz, DMSO- d 6 ): δ =6.18 (m, 1H), 6.43 (ddd, J HH =8.2, 6.7, 1.1 Hz, 1H), 6.66 (m, 1H), 6.73–6.79 (m, 3H), 7.07 (pt, 1H), 7.22–7.31 (m, 2H), 7.36–7.40 (m, 4H), 7.50–7.59 (m, 5H), 7.80 (d, J HH =7.2 Hz, 2H), 7.97 (d, J HH =8.3 Hz, 1H), 9.02 (s, 1H). 13 C NMR (125 MHz, DMSO- d 6 ): δ =114.58, 115.69, 116.33, 121.54, 121.87, 123.04, 123.38, 125.86, 126.69, 126.95, 127.63, 128.97, 129.22, 129.27, 130.06, 133.30, 133.97, 134.61, 135.11, 136.81, 138.36, 143.26, 143.64, 156.01, 162.46, 166.61, 169.69. MS (MALDI+) m/z found 524.2 ([M + ]), calcd. 524.1. Elemental analysis calcd. (%) for C 32 H 22 N 2 NiO 2 ·AcO − ·2H 2 O C 65.83, H 4.71, N 4.52 found C 65.50, H 4.71, N 4.52. For 1 H NMR and 13 C{ 1 H} DEPT spectra see Supplementary Fig. S21 . Synthesis of Bis-Schiff base ligand 3 ( E )-2-(((2-aminophenyl)imino) (phenyl)methyl) phenol (100 mg, 0.35 mmol) and 3,3′-diformyl-2,2′-dihydroxy-1,1′- biphenyl (93 mg, 0.38 mmol) were dissolved in 5 ml of MeOH and stirred for 18 h. A yellow suspension was formed, the solid was filtered and washed with methanol. Yellow solid, 189 mg, 97%. 1 H NMR (400 MHz, CDCl 3 ): δ =6.73 (m, 2H), 6.82 (m, 1H), 6.98–7.09 (m, 9H), 7.20 (m, 2H), 7.36 (m, 2H), 7.49 (dd, J HH =7.5, 1.5 Hz, 1H), 7.57 (ddd, J HH =12.5, 7.5, 1.5 Hz, 1H), 8.39 (s, 1H), 9.94 (s, 1H), 11.16 (s, 1H), 13.57 (s, 1H), 14.07 (s, 1H). 13 C NMR (100 MHz, CDCl 3 ): δ =118.05, 118.12, 118.65, 119.15, 119.57, 119.61, 119.70, 121.21, 123.39, 124.91, 125.67, 126.47, 127.07, 128.00, 128.69. 129.10, 132.42, 132.50, 133.15, 133.56, 134.67, 135.43, 139.23, 139.84, 141.58, 159.14, 159.31, 162.80, 163.09, 174.96, 196.45. HRMS (ES+) m/z found 513.1798 ([M + H]), C 33 H 25 N 2 O 4 requires 513.1814. For 1 H NMR and 13 C{ 1 H} DEPT spectra see Supplementary Fig. S22 . Synthesis of Bis-Schiff base Zn complex 3a A solution of 3 (100 mg, 0.2 mmol) in 3 ml of CH 2 Cl 2 and Zn(AcO) 2 ·2 H 2 O (50 mg, 0.23 mmol) in 5 ml of MeOH was stirred for 18 h. A yellow suspension was formed, the solid was filtered and washed with methanol. Bright yellow solid, 120 mg, 99%. 1 H NMR (400 MHz, DMSO- d 6 ): δ =6.29 (t, J HH =7.6 Hz, 2H), 6.53 (d, J HH =8.0 Hz, 1H), 6.74 (d, J HH =8.5 Hz, 1H), 6.89 (dd, J HH =13.7, 7.9 Hz, 3H), 7.07 (t, J HH =7.5 Hz, 1H), 7.16 (m, 2H), 7.28 (m, 2H), 7.41 (m, 3H), 7.55 (d, J HH =7.1 Hz, 1H), 7.63 (d, J HH =7.9 Hz, 1H), 7.68 (t, J HH =6.4 Hz, 3H), 9.03 (s, 1H), 10.64 (s, 1H), 11.77 (s, 1H). 13 C NMR (125 MHz, DMSO- d 6 ): δ =112.40, 115.98, 117.47, 119.71, 120.42, 120.94, 123.29, 124.39, 125.09, 125.89, 125.95, 126.42, 128.22, 128.50, 128.63, 130.80, 131.18, 133.42, 134.38, 136.62, 136.71, 136.80, 137.27, 139.57, 139.82, 160.63, 163.51, 165.44, 172.37, 173.94, 190.75. MS (MALDI+) m/z found 575.1 ([M + ]), calcd. 574.1. Elemental analysis calcd. (%) for C 33 H 22 N 2 O 4 Zn·5MeOH C 62.00, H 5.75, N 3.81 found C 62.30, H 4.73, N 3.97. For 1 H NMR and 13 C{ 1 H} DEPT spectra see Supplementary Fig. S23 . For X-ray crystallographic structure see Supplementary Fig. S24 . Synthesis of Bis-Schiff base Ni complex 3b A solution of 3a (50 mg, 0.087 mmol) in 7 ml of THF and Ni(AcO) 2 ·4H 2 O (22.7 mg, 0.091 mmol) in 2.5 ml of THF was stirred for 18 h. Solvent was the evaporated and the brownish solid washed with MeOH. Brown solid, 49 mg, 98%. 1 H NMR (500 MHz, CDCl 3 ): δ =6.07 (d, J HH =8.3 Hz, 1H), 6.40 (pt, JHH=7.2 Hz, 1H), 6.55 (pt, JHH=7.0 Hz, 1H), 6.81 (m, 3H), 6.89 (pt, J HH =7.2 Hz, 1H), 7.06 (pt, J HH =7.0 Hz, 1H), 7.16 (m, 3H), 7.39–7.51 (m, 6H), 7.60 (d, J HH =7.0 Hz, 1H), 7.80 (d, J HH =7.1 Hz, 1H), 8.16 (s, 1H), 9.81 (s, 1H)10.64 (s, 1H). 13 C NMR (1250 MHz, CDCl 3 ): δ =114.87, 115.30, 117.36, 120.31, 121.33, 122.13, 123.47, 124.04, 125.65, 126.61, 128.44, 129.03, 129.28, 129.69, 129.99, 130.21, 133.56, 134.23, 134.98, 136.68, 138.17, 138.41, 143.41, 144.80, 154.44, 160.11, 160.71, 166.72, 169.79, 169.89, 192.97. MS (MALDI+) m/z found 568.2 ([M + ]), calcd. 568.1. Elemental analysis calcd. (%) for C 33 H 22 N 2 NiO 4 ·5H 2 O C 60.12, H 4.89, N 4.25 found C 60.41, H 3.55, N 4.07. For 1 H NMR and 13 C{ 1 H} DEPT spectra see Supplementary Fig. S25 . Synthesis of Tetrakis–Schiff base ligand 5 ( E )-2-(1-((2-aminophenyl) imino)-ethyl) phenol (500 mg, 2.2 mmol) and 3,3′-diformyl-2,2′-dihydroxy-1,1′- biphenyl (267 mg, 1.1 mmol) were dissolved in 10 ml of MeOH and the solution was stirred for 18 h. The precipitate formed was then filtered. Yellow solid, 581 mg, 80%. 1 H NMR (500 MHz, CDCl 3 ): δ =2.23 (s, 6H, CH 3 ), 6.83 (m, 4H, CH phen , J HH =8, J HH =4.2), 6.96 (pt, 4H, CH ar , J HH =9.6, J HH =4.2), 7.27 (m, 10H, CH ar ), 7.35 (dd, 2H, CH phen , J HH =8, J HH =1.4), 7.55 (dd, 2H, CH phen , J HH =8, J HH =1.4), 8.62 (s, CH imine , 2H), 13.11 (s, OH ald , 2H), 14.23 (s, OH ket , 2H). 13 C NMR (125.5 MHz, CDCl 3 , 298 K): δ = = 18.20, 118.13, 118.26, 118.48, 119.47, 119.70, 119.83, 122.49, 125.27, 125.94, 127.40, 129.26, 131.99, 133.14, 135.99, 140.11, 141.20, 158.80, 162.05, 163.75, 172.59. HRMS (MALDI +) m/z 659.2515 ([M + H]) C 42 H 34 N 4 O 4 requires 659.7517. For 1 H NMR and 13 C{ 1 H} DEPT spectra see Supplementary Fig. S26 . Synthesis of Tetrakis–Schiff base Zn complex 5a To a solution of 5 (200 mg, 0.3 mmol) in 20 ml of anhydrous THF, ZnEt 2 (0.72 ml 1 M in hexanes, 0.72 mmol) were slowly added. The reaction was stirred at room temperature over night. The yellow precipitate was filtered. Yellow solid, 240 mg, 99%. 1 H NMR (400 MHz, DMSO- d 6 , 298 K): δ =2.48 (s, 6H, CH 3 ), 6.82 (m, 2H), 6.41 (pt, 2H), 6.54 (pd, 2H), 7.00 (m, 2H), 7.21 (d, 2H), 7.33 (m, 4H), 7.42 (d, 2H), 7.67 (dd, 4H), 8.92 (s, 2H, CH ald ). 13 C NMR (75 MHz, DMSO- d 6 , 298 K): δ =112.13, 112.63, 117.15, 119.42, 123.15, 123.41, 123.93, 124.22, 125.60, 126.62, 131.12, 132.13, 134.75, 136.83, 139.34, 140.00, 163.57, 167.89, 171.18, 173.09. MS (MALDI +) m/z found 786.2 ([M + H]), calcd. 784.1. Elemental analysis calcd. (%) for C 42 H 30 N 4 O 4 Zn 2 ·10H 2 O: C 52.24, H 5.22, N 5.80 found C 52.64, H 3.78, N 5.48. For 1 H NMR and 13 C{ 1 H} DEPT spectra see Supplementary Fig. S27 . Synthesis of Tetrakis–Schiff base Ni complex 5b To a solution of 5a (50 mg, 0.06 mmol) in 6 ml of THF, 2 equivalents of Ni(AcO) 2 ·4H 2 O were added. The reaction was stirred 18 h and the brown solid filtered and washed with MeOH. Brown solid, 45 mg, 92%. 1 H NMR (500 MHz, DMSO- d 6 , 298 K): δ =1.24 (s, 6H, CH 3 ), 6.30 (m, 2H), 6.60 (t, 2H, J HH =8.23, 7.90 Hz), 6.65 (d, 4H, J HH =3.67 Hz), 7.13 (t, 2H, J HH =7.95, 1.07 Hz), 7.24 (t,H, J HH =8.38, 1.07 Hz), 7.29 (dd, 2H, J HH =8.16, 1.07 Hz), 7.38 (dd, 2H, J HH =7.09, 1.93 Hz), 7.40 (d, 2H, J HH =8.38 Hz), 7.45 (dd, 2H, J HH =8.16, 1.93), 8.02 (dd, 2H, J HH =8.37, 0.97 Hz), 8.70 (s, CH ald ). MS (MALDI +) m/z found 770.3 ([M + ]), calcd. 770.1. Elemental analysis calcd. (%) for C 42 H 30 N 4 Ni 2 O 4 ·8H 2 O·3MeOH: C 53.39, H 4.77, N 5.53 found C 53.24, H 4.26, N 5.26. For 1 H NMR spectra see Supplementary Fig. S28 . Accession codes: The X-ray crystallographic coordinates for structures reported in this Article have been deposited at the Cambridge Crystallographic Data Centre (CCDC), under deposition numbers CCDC 936467, 936468 and 936469 (see Supplementary Data 1–3 ). These data can be obtained free of charge from The Cambridge Crystallographic Data Centre via www.ccdc.cam.ac.uk/data_request/cif . How to cite this article: Escárcega-Bobadilla, M. V. et al. Nanorings and rods interconnected by self-assembly mimicking an artificial network of neurons. Nat. Commun. 4:2648 doi: 10.1038/ncomms3648 (2013).